Rab9 and retromer regulate retrograde trafficking of luminal protein required for epithelial tube length control Apical extracellular matrix filling the lumen controls the morphology and geometry of epithelial tubes during development, yet the regulation of luminal protein composition and its role in tube morphogenesis are not well understood. Here we show that an endosomal-retrieval machinery consisting of Rab9, retromer and actin nucleator WASH (Wiskott–Aldrich Syndrome Protein and SCAR Homolog) regulates selective recycling of the luminal protein Serpentine in the Drosophila trachea. Secreted Serpentine is endocytosed and sorted into the late endosome. Vps35, WASH and actin filaments differentially localize at the Rab9-enriched subdomains of the endosomal membrane, where Serpentine containing vesicles bud off. In Rab9, Vps35 and WASH mutants, Serpentine was secreted normally into the tracheal lumen, but the luminal quantities were depleted at later stages, resulting in excessively elongated tubes. In contrast, secretion of many luminal proteins was unaffected, suggesting that retrograde trafficking of a specific class of luminal proteins is a pivotal rate-limiting mechanism for continuous tube length regulation. Tubular organs support the uptake and exchange of nutrition, metabolites and gases that are essential for the normal physiology of animals. During development, geometry of such tubes must be precisely controlled, so that the circulation of luminal components matches the size of the growing organ and the rest of the organism. Loss of tube size regulation leads to pathological tubule dysfunctions such as polycystic kidney disease [1] . The Drosophila tracheal system is a well-characterized model system for tubular organ morphogenesis [2] , [3] , [4] , [5] . After tube connection is complete, tracheal tubes undergo diametric and axial expansion to reach their final shape without cell proliferation, followed by clearance of luminal contents and gas filling before the larvae hatch into an air-filled environment [6] . Tracheal diametric expansion is initiated by a cell-intrinsic programme of apical membrane growth and secretion of luminal materials [7] , including zona pellucida domain-containing protein Piopio (Pio) and 2A12 antigen driven by the actin nucleator Dia and Myosin V motor [6] , [8] , and chitin, the major component of the apical extracellular matrix (aECM). Deposition of those luminal materials promotes the rapid diametric expansion [9] , [10] , [11] . Longitudinal-axial growth follows diametric expansion. Src kinase has been recently identified as a positive factor for tube elongation [12] , [13] . aECM acts as a negative factor required to restrict tube length to a proper level [14] . When the remodelling of chitin polymer is compromised due to mutation of the secreted chitin deacetylases Serpentine (Serp) and Vermiform (Verm), the tracheal tubules exceed normal length [15] , [16] . Thus, maintaining the proper chitin deacetylase level is important for tube-length determination. The luminal localization of Serp and Verm is independent of Dia and Myosin V [8] . Thus, how chitin-modification enzymes are maintained in the tube and how cells dynamically regulate extracellular matrix protein composition in the lumen are not understood. Retrograde protein trafficking involves the sorting of endocytosed proteins into a tubular endosomal membrane, which buds off and then fuses with the trans -Golgi network (TGN) [17] , [18] . This pathway requires the endosomal Rab family GTPase Rab9 (refs 19 , 20 , 21 , 22 ), the retromer, a multiple protein complex required for the outward budding of the endosomal membrane [23] , [24] , [25] , [26] and actin nucleation-promoting factors WASH (Wiskott–Aldrich Syndrome Protein and SCAR Homolog) [27] , [28] . The protein cargoes recycled in this pathway include Mannose 6-phosphate receptors [19] , [23] , cell-surface protein Crumbs (Crb) [29] , [30] and Wntless/Sprinter/Evenness [31] , [32] , [33] , [34] , [35] . The key remaining question is whether this pathway acts beyond the role in constitutive protein turnover and has an active regulatory role in morphogenesis. Here we addressed the role of retrograde trafficking in tracheal tube morphogenesis, and found that Rab9, Vps35 (the core component of the retromer’s cargo recognition complex) and WASH together control the tracheal tube length by positively regulating the luminal deposition of Serp. We further show that Serp is a specific cargo for retromer-dependent endocytic trafficking. Combining genetic, biochemical and cell biological approaches, we established the relationship between Rab5, Rab9 and Rab7 in the retromer recruitment, and propose that Rab9 and the retromer function cooperatively in endocytotic Serp sorting from late endosomes (LEs) to the TGN via a WASH-associated vesicle-budding machinery. Our study further elucidates the connection between luminal protein trafficking and epithelial tube size control. Requirement for Rab9 in tracheal tube length restriction Rab9 was identified from a screen of Rab family proteins showing localization similar to Arf-like3 GTPase in the tracheal system [36] . Rab9 mRNA was detected broadly in embryonic tissues, including the tracheal system (white arrowhead in Supplementary Fig. S1a ). Three lethal deletions of rab9 were identified by mobilization of Minos transposon [37] inserted into the rab9 locus ( Supplementary Fig. S1c ). In situ hybridization demonstrated that the mRNA expression level was significantly decreased in rab9 -mutant homozygous embryos compared with wild-type embryos ( Supplementary Fig. S1a,b ). Trans-heterozygosity of rab9 56 and rab9 199 created a deletion of rab9 only, and was used to identify rab9 -mutant phenotypes. The most apparent defect among rab9 mutants ( rab9 56 / rab9 199 and homozygotes of each mutant) was a convoluted dorsal trunk (DT) that was increased in length by approximately 15%, compared with wild-type embryos ( Fig. 1a , Supplementary Fig. S1d–f ). In contrast, the tube diameter was unaffected by the mutations ( Supplementary Fig. S1g ). Expression of UAS-GFP-Rab9 in the trachea (with btl -Gal4 driver) in rab9 mutants rescued the tracheal tube phenotype ( Fig. 1c ), indicating that Rab9 is essential for restricting the tracheal tube length. 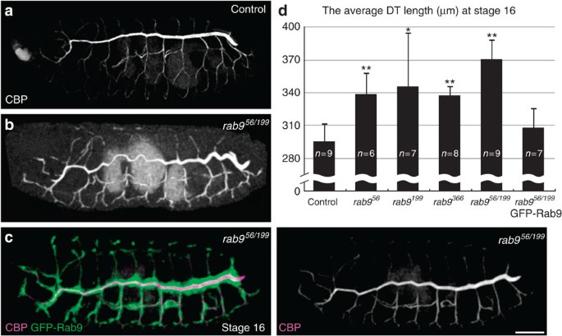Figure 1: Requirement of Rab9 for tracheal tube length restriction. (a–c)rab9-mutant phenotype. Stage-16 controlrab956/+ embryo (a),rab956/rab9199-mutant (b) andrab956/rab9199-mutant embryos expressing GFP-Rab9 in the trachea (withbtl-Gal4 driver) (c) labelled with a fluorescent CBP to reveal tube lumen. (d) Quantification of the DT length in control andrab9-mutant embryos at stage 16. Error bars represent s.d. The single and double asterisks representP<0.05 and 0.001<P<0.01, respectively, compared with the control by Student’st-test (n=6–9 embryos). Scale bar, 50 μm. Figure 1: Requirement of Rab9 for tracheal tube length restriction. ( a – c ) rab9 -mutant phenotype. Stage-16 control rab9 56 /+ embryo ( a ), rab9 56 /rab9 199 -mutant ( b ) and rab9 56 /rab9 199 -mutant embryos expressing GFP-Rab9 in the trachea (with btl -Gal4 driver) ( c ) labelled with a fluorescent CBP to reveal tube lumen. ( d ) Quantification of the DT length in control and rab9 -mutant embryos at stage 16. Error bars represent s.d. The single and double asterisks represent P <0.05 and 0.001< P <0.01, respectively, compared with the control by Student’s t -test ( n =6–9 embryos). Scale bar, 50 μm. Full size image Rab9 is required for the luminal retention of Serp The long tracheal tube phenotype of the rab9 mutants resembled that of chitin deacetylase mutants [15] , [16] . The secreted chitin deacetylase Serp was first detected as cytoplasmic puncta in tracheal cells; it was then released into the lumen at the onset of the massive secretion that initiates tube diameter expansion ( Supplementary Fig. S2a ) [6] . At this stage, the GFP-Rab9 puncta overlapped only minimally with Serp ( Fig. 2c and Supplementary Fig. S2a,b ). After stage 15, the Serp-positive fraction among the GFP-Rab9 endosomes increased while the tracheal lumen expansion proceeded ( Fig. 2a–c ). A similar colocalization of RFP-Rab9 and Serp-chitin-binding domain (CBD)-GFP [15] was observed in the tracheal system, in which Serp puncta were contained within RFP-Rab9 endosomes ( Fig. 2d ). 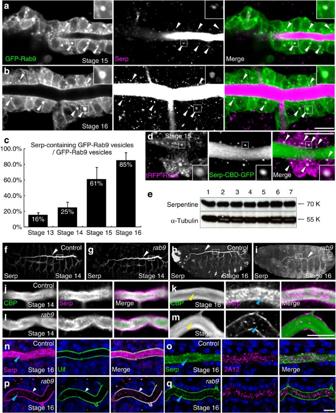Figure 2: Rab9 regulates endocytic recycling of Serp. (a–c) Colocalization of GFP-Rab9 and Serp in the tracheal cells at late stages of embryogenesis (stages 15 and 16, white arrowheads ina,b). Insets inaandbshow GFP-Rab9 endosomes containing Serp. The colocalization rate increased as development proceeded (c). (d) Tracheal cells expressing RFP-Rab9 and Serp-chitin-binding domain-GFP (Serp-CBD-GFP) driven bybtl-GAL4, showing colocalization of the two markers (arrowheads). Inset shows enlargement of endosome. (e) Western blotting of whole-cell lysates from 20 embryos probed with anti-Serp antibody. 1,btl-GAL4>GFP-Rab9; 2, Df(2L) Exel8041/+; 3, Df(2L)Exel8041 homozygote; 4,rab956/+; 5,rab956homozygote; 6,rab9199/+; and 7,rab9199homozygote. (f–m) Control heterozygotes (f,h) andrab956/rab9199(g,i) embryos at stage 14 and 16 were immunostained with Serp and CBP. White arrowheads inf–ishow the expression level of Serp in tracheal tubes inrab9-mutant embryos was unaltered at stage 14 (j,l) and apparently decreased at stage 16 (k,m) compared with control embryos. Blue arrowheads (k,m,n–q) show the significant reduction of Serp protein in therab9-mutant tracheal lumen, whereas the chitin expression showed no difference between the control andrab9-mutant embryo (yellow arrowheads ink,m). (n,p) Stage-16rab9-mutant heterozygous (n) and homozygous (p) embryos immunostained for Serp and Uninflatible (Uif). White arrowheads inpshow Serp colocalized with apical membrane marker Uif. (o,q) Stage-16rab9-mutant heterozygous (o) and homozygous (q) embryos immunostained for Serp and 2A12 antigen. Blue arrowheads show Serp significantly decreased in the lumen, but 2A12 does not show detectable difference betweenrab9mutant and the control. Scale bar, 10 μm. Figure 2: Rab9 regulates endocytic recycling of Serp. ( a – c ) Colocalization of GFP-Rab9 and Serp in the tracheal cells at late stages of embryogenesis (stages 15 and 16, white arrowheads in a , b ). Insets in a and b show GFP-Rab9 endosomes containing Serp. The colocalization rate increased as development proceeded ( c ). ( d ) Tracheal cells expressing RFP-Rab9 and Serp-chitin-binding domain-GFP (Serp-CBD-GFP) driven by btl -GAL4, showing colocalization of the two markers (arrowheads). Inset shows enlargement of endosome. ( e ) Western blotting of whole-cell lysates from 20 embryos probed with anti-Serp antibody. 1, btl -GAL4>GFP-Rab9; 2, Df(2L) Exel8041/+; 3, Df(2L)Exel8041 homozygote; 4, rab9 56 /+; 5, rab9 56 homozygote; 6, rab9 199 /+; and 7, rab9 199 homozygote. ( f – m ) Control heterozygotes ( f , h ) and rab9 56 /rab9 199 ( g , i ) embryos at stage 14 and 16 were immunostained with Serp and CBP. White arrowheads in f – i show the expression level of Serp in tracheal tubes in rab9 -mutant embryos was unaltered at stage 14 ( j , l ) and apparently decreased at stage 16 ( k , m ) compared with control embryos. Blue arrowheads ( k , m , n – q ) show the significant reduction of Serp protein in the rab9 -mutant tracheal lumen, whereas the chitin expression showed no difference between the control and rab9 -mutant embryo (yellow arrowheads in k , m ). ( n , p ) Stage-16 rab9 -mutant heterozygous ( n ) and homozygous ( p ) embryos immunostained for Serp and Uninflatible (Uif). White arrowheads in p show Serp colocalized with apical membrane marker Uif. ( o , q ) Stage-16 rab9 -mutant heterozygous ( o ) and homozygous ( q ) embryos immunostained for Serp and 2A12 antigen. Blue arrowheads show Serp significantly decreased in the lumen, but 2A12 does not show detectable difference between rab9 mutant and the control. Scale bar, 10 μm. Full size image In rab9 -mutant embryos, Serp secretion at early stage (stage 14) was normal ( Fig. 2f ). At late stage (stage 16), Serp expression was reduced in the tracheal lumen (blue arrowheads in Fig. 2k ), and the Serp associated with the apical membrane was increased ( Fig. 2p , white arrowheads). Strikingly, chitin deposition was not altered in rab9 mutants (compare Fig. 2m with Fig. 2k , yellow arrowheads). To determine whether other luminal or membrane proteins were affected, we examined the expression and localization of the luminally accumulated 2A12 antigen ( Fig. 2o ), Pio and Verm ( Supplementary Fig. S2c,d ) and the membrane proteins Crb and Uninflatible (Uif) ( Supplementary Fig. S2e,f ), and found that their expression and localization were unaltered in the rab9 mutants. These data indicated that among the luminal and membrane proteins examined, Serp specifically requires Rab9 for its luminal localization. To learn whether Rab9 is involved in the protein stability of Serp, we examined the expression level of Serp by western blotting, and found that the total amount of Serp was not altered by the rab9 mutation ( Fig. 2e ), suggesting that Rab9 regulates the localization rather than the stability of Serp. Rab9 is involved in trafficking from endosomes to the TGN To determine if Rab9 is involved in endocytic trafficking, we conducted a dextran dye uptake assay using fly embryos ( Fig. 3a ). The labelled dextran was found associated with GFP-Rab9 endosomes (arrowheads in Fig. 3a ) at 30 min after dye injection and co-trafficked in tracheal cells ( Fig. 3b ). In S2 cells, the labelled dextran was included in GFP-Rab9-labelled vacuoles ( Fig. 3c ), indicating that Rab9 is involved in endocytic trafficking. Because Rab9 is implicated in retrograde trafficking in vitro [19] , [20] , we predicted that Rab9 would be colocalized with the TGN or the early or late endosomal markers. To test this hypothesis, we expressed markers for the TGN (GalT-CFP), early endosomes (GFP-Rab5), LEs (YFP-Rab7), lysosomes (GFP-LAMP1) or endoplasmic reticulum (GFP-KDEL) in RFP-Rab9-expressing tracheal cells. We found that RFP-Rab9 colocalized with GalT-CFP, GFP-Rab5 and YFP-Rab7 (blue arrowheads in Fig. 3d–f ). Partial colocalization was observed with GFP-LAMP1 ( Fig. 3g ), but not with GFP-KDEL ( Fig. 3h ). The recycling endosome marker Rab11 did not colocalize with GFP-Rab9 ( Fig. 3i ). Collectively, these results suggest that Rab9 is involved in the trafficking pathway from endosomes to the TGN. 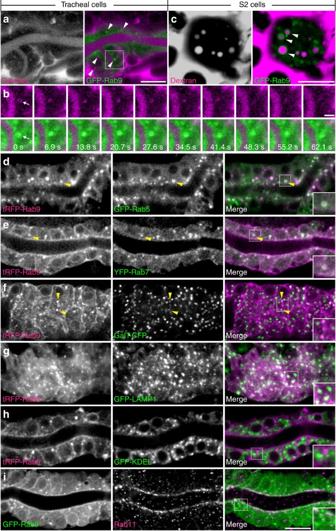Figure 3: Rab9 is involved in the trafficking pathway from endosomes to the TGN. (a–c) Confocal images of dextran-injected embryos (a,b) and S2 cells (c) expressing GFP-Rab9. White arrowheads inaandcindicate the endocytic dextran puncta surrounded by GFP-Rab9 at 30 min after dye injection. The boxed region inawas observed by time-lapse imaging, which shows the co-trafficking of the dextran and GFP-Rab9 signals (white arrows inb). (d–i) Subcellular localization of fluorescent protein-fused Rab9 in the tracheal cells. Stage 16 embryos co-expressing RFP-Rab9 with GFP-Rab5 (d), YFP-Rab7 (e), GalT-CFP (f), GFP-LAMP1 (g) and GFP-KDEL (h) driven bybtl-GAL4. (i) Confocal images of the tracheal cells expressing GFP-Rab9 and immunostained with Rab11 antibody. Insets ind,e,fandgshow RFP-Rab9 endosomes colocalized with early endosomes, LEs and TGN markers, respectively, and partially colocalized with the lysosome marker (g). No colocalization of fluorescent Rab9 with endoplasmic reticulum (h) or the recycling endosome marker (i) was observed. Scale bar, 2 μm forband 10 μm fora,c–i. Figure 3: Rab9 is involved in the trafficking pathway from endosomes to the TGN. ( a – c ) Confocal images of dextran-injected embryos ( a , b ) and S2 cells ( c ) expressing GFP-Rab9. White arrowheads in a and c indicate the endocytic dextran puncta surrounded by GFP-Rab9 at 30 min after dye injection. The boxed region in a was observed by time-lapse imaging, which shows the co-trafficking of the dextran and GFP-Rab9 signals (white arrows in b ). ( d – i ) Subcellular localization of fluorescent protein-fused Rab9 in the tracheal cells. Stage 16 embryos co-expressing RFP-Rab9 with GFP-Rab5 ( d ), YFP-Rab7 ( e ), GalT-CFP ( f ), GFP-LAMP1 ( g ) and GFP-KDEL ( h ) driven by btl -GAL4. ( i ) Confocal images of the tracheal cells expressing GFP-Rab9 and immunostained with Rab11 antibody. Insets in d , e , f and g show RFP-Rab9 endosomes colocalized with early endosomes, LEs and TGN markers, respectively, and partially colocalized with the lysosome marker ( g ). No colocalization of fluorescent Rab9 with endoplasmic reticulum ( h ) or the recycling endosome marker ( i ) was observed. Scale bar, 2 μm for b and 10 μm for a , c – i . Full size image Vps35 regulates Serp-dependent tracheal tube-length control The results described above are consistent with a model in which Rab9 has a role in the recycling of Serp from endosomes to the TGN. To determine if the retromer complex is involved in this process, we first examined the tracheal tube phenotype in zygotic mutants of vps35 (core retromer component). vps35 [31] exhibited the long-tube phenotype ( Fig. 4a ) and reduced luminal Serp levels ( Fig. 4f and Supplementary Fig. S3a,b ). The luminal labelling of 2A12, chitin-binding probe (CBP) and Pio was unaffected ( Supplementary Fig. S3a–d ). This phenotype was identical to that observed in the rab9 mutants. In addition, a mild reduction in Crb expression was noted ( Supplementary Fig. S3e,f ), as previously described for maternal vps35 mutants [30] . A combination of the vps35 and rab9 mutants did not exacerbate the mutant phenotypes ( Fig. 4c–e ), suggesting that vps35 and rab9 act in the same genetic pathway. 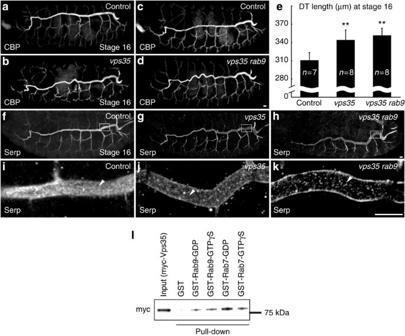Figure 4: Vps35 works together with Rab9 for Serp trafficking and tracheal tube length control. (a–d) Control heterozygote (a,c),vps351(b) andvps351rab956/vps351rab9199(d) embryos at stage 16 stained with CBP. (e) Quantification of DT length. Double (**) asterisks represent a significant difference from the control by Student’st-test (0.001<P<0.01). (f–k) Embryos immunostained with the Serp antibody. White arrowheads indicate Serp signal in the DT lumen. (l) Rab9 interacts with Vps35 in GST pull-down assay. Immobilized GST, GST-Rab9 and GST-Rab7 were conversed into GDP (inactive) and GTP (active) forms, respectively, then loaded with extract of S2 cells expressing myc-Vps35. The bound protein complex were detected by anti-myc antibody. Input represent 3% of the loaded extract. Scale bar, 10 μm. Figure 4: Vps35 works together with Rab9 for Serp trafficking and tracheal tube length control. ( a – d ) Control heterozygote ( a , c ), vps35 1 ( b ) and vps35 1 rab9 56 /vps35 1 rab9 199 ( d ) embryos at stage 16 stained with CBP. ( e ) Quantification of DT length. Double (**) asterisks represent a significant difference from the control by Student’s t -test (0.001< P <0.01). ( f – k ) Embryos immunostained with the Serp antibody. White arrowheads indicate Serp signal in the DT lumen. ( l ) Rab9 interacts with Vps35 in GST pull-down assay. Immobilized GST, GST-Rab9 and GST-Rab7 were conversed into GDP (inactive) and GTP (active) forms, respectively, then loaded with extract of S2 cells expressing myc-Vps35. The bound protein complex were detected by anti-myc antibody. Input represent 3% of the loaded extract. Scale bar, 10 μm. Full size image Vps35 interacts with Rab9 in Drosophila S2 cells As both Rab9 and Vps35 are required for Serp trafficking and may act in the same genetic pathway, we next examined whether Rab9 and Vps35 can physically interact each other. The purified GST-Rab9 were immobilized on glutathione-sepharose beads and conversed into guanosine diphosphate (GDP)- and guanosine triphosphate (GTP)-loaded forms. Then myc-Vps35 lysates from S2 cells was loaded onto the samples, and the detected results showed that both GTP- and GDP-loaded forms of GST-Rab9, but not GST pulled down myc-Vps35 ( Fig. 4l ), indicating that Rab9 physically interacts with Vps35. Similar interaction was observed with GST-Rab7. Vps35 and Serp colocalize at late endosomal Rab9 domains The binding of Rab9 with Vps35 prompted us to further examine their endosomal localization in S2 cell and the tracheal system. When Vps35-mRFP was coexpressed with GFP-Rab9 in S2 cells, the Vps35-mRFP signal was detected as small puncta localized to small endosomes and vacuolar endosomes labelled with GFP-Rab9 ( Fig. 5a , yellow and white arrowhead). Moreover, the Vps35-mRFP signal coincided with the enrichment of GFP-Rab9 in the vacuolar endosomal membrane ( Fig. 5c and white arrowheads in Fig. 5a ), implying that the retrieval vesicles formed at these domains. In GFP-Rab9- and myc-DVps35-expressing tracheal cells, Vps35 also localized at the Rab9-labelling endosomal membrane (white arrowheads in the insets in Fig. 5e ). Consistent with this finding, time-lapse observation of GFP-Rab9 revealed small vesicles budding off the Rab9 endosomes within 40–50 s ( Fig. 5d and Supplementary Movie 1 ). Long tubular structures were often observed in GFP-Rab7 and RFP-Rab9 co-expressing endosomal membrane (yellow arrowheads in Fig. 5i ). Knockdown of Vps35 compromised this phenotype ( Fig. 5j ), indicating that Vps35 is required for the tubular structure formation. 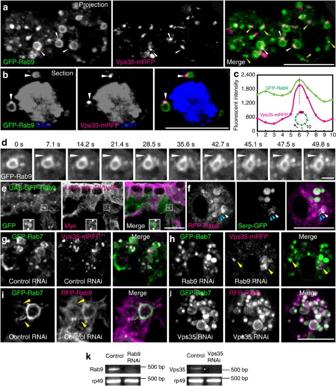Figure 5: Vps35 and Serp colocalize at Rab9-enriched domains in the late-endosome membrane. (a,b) S2 cells expressing GFP-Rab9 and Vps35-mRFP. Yellow and white arrowheads show the colocalization of Vps35-mRFP with GFP-Rab9-enriched membrane domains of small endosomes and vacuolar endosome, respectively. (c) Fluorescent intensity of GFP-Rab9 (green) and Vps35-mRFP (magenta) in an endosomal membrane. (d) Budding of GFP-Rab9 endosomes in S2 cells. White arrowheads indicate small vesicle formation, budding and release from the endosome (Supplementary Movie 1). (e) Tracheal cells co-expressing GFP-Rab9 and myc-Vps35. White arrowheads in the insets indicate myc-Vps35 puncta localized on the Rab9 endosomal membrane. (f) Colocalization of Serp-GFP with RFP-Rab9 in S2 cells. White arrowheads indicate that the Serp-GFP colocalizes with RFP-Rab9 in the endosomal membrane. Blue arrowheads indicate the colocalization of Serp-GFP puncta with small RFP-Rab9 vesicles in the cytoplasm. (g,h) S2 cells were co-transfected with GFP-Rab7 and Vps35-mRFP, then treated with control (g) and Rab9 (h) dsRNA. (i,j) S2 cells were co-transfected with GFP-Rab7 and RFP-Rab9, then treated with control (i) and Vps35 (j) dsRNA. Yellow arrowheads in (i) showed the tubule structures extending from endosomes. (k) Reverse transcription PCR of Rab9 and Vps35 fragment from the control and dsRNA-treated cells. rp49 was amplified for the internal control. Scale bar, 10 μm fora,bande–jand 2 μm ford. Figure 5: Vps35 and Serp colocalize at Rab9-enriched domains in the late-endosome membrane. ( a , b ) S2 cells expressing GFP-Rab9 and Vps35-mRFP. Yellow and white arrowheads show the colocalization of Vps35-mRFP with GFP-Rab9-enriched membrane domains of small endosomes and vacuolar endosome, respectively. ( c ) Fluorescent intensity of GFP-Rab9 (green) and Vps35-mRFP (magenta) in an endosomal membrane. ( d ) Budding of GFP-Rab9 endosomes in S2 cells. White arrowheads indicate small vesicle formation, budding and release from the endosome ( Supplementary Movie 1 ). ( e ) Tracheal cells co-expressing GFP-Rab9 and myc-Vps35. White arrowheads in the insets indicate myc-Vps35 puncta localized on the Rab9 endosomal membrane. ( f ) Colocalization of Serp-GFP with RFP-Rab9 in S2 cells. White arrowheads indicate that the Serp-GFP colocalizes with RFP-Rab9 in the endosomal membrane. Blue arrowheads indicate the colocalization of Serp-GFP puncta with small RFP-Rab9 vesicles in the cytoplasm. ( g , h ) S2 cells were co-transfected with GFP-Rab7 and Vps35-mRFP, then treated with control ( g ) and Rab9 ( h ) dsRNA. ( i , j ) S2 cells were co-transfected with GFP-Rab7 and RFP-Rab9, then treated with control ( i ) and Vps35 ( j ) dsRNA. Yellow arrowheads in ( i ) showed the tubule structures extending from endosomes. ( k ) Reverse transcription PCR of Rab9 and Vps35 fragment from the control and dsRNA-treated cells. rp49 was amplified for the internal control. Scale bar, 10 μm for a , b and e – j and 2 μm for d . Full size image We next followed the vesicular movement of full-length Serp-GFP, and found that it was associated with the Rab9-positive endosomal membrane, and some of the Serp-GFP was concentrated at the Rab9-enriched domains (white arrowheads in Fig. 5f ). Importantly, the Serp puncta colocalized with small GFP-Rab9 vesicles that were budding from larger endosomes (blue arrowheads in Fig. 5f ). Endosomal recruitment and sorting of Vps35 We next asked the role of Rab proteins in endosomal recruitment of Vps35. We observed the colocalization of GFP-Rab5 and RFP-Rab9 in tracheal cells ( Fig. 3d ). In S2 cells ( Supplementary Fig. S4a ), they colocalized in two populations. One is large vacuoles where localization of GFP-Rab5 was weaker compared with RFP-Rab9, or transient ( Supplementary Fig. S4a–c , Supplementary Movie 2 ). The other is small vesicles with high GFP-Rab5 concentration (diameter <0.4 μm, Supplementary Fig. S4a–c ). Decrease of Rab5 expression by RNA interference (RNAi) treatments reduced vacuolar population of RFP-Rab9 and dissociation of Vps35-mRFP from endosomal membrane ( Supplementary Fig. S4d,e , see also similar results by expression of the GDP-locked from GFP-Rab5-S43N, Supplementary Fig. S4h,i ), suggesting that Rab5 is essential for recruitment of Vps35 and maturation of Rab9 LE. Downregulation of Rab9 expression using RNAi treatment caused dissociation of Vps35-mRFP puncta from vacuolar LEs (yellow arrowheads in Fig. 5h , compared with Fig. 5g ). On the other hand, overexpression of a GDP-locked form GFP-Rab9-S26N caused Vps35-mRFP to spread on the entire vacuolar membrane (white arrowheads in Supplementary Fig. S4j ). Given the result of Vps35 association with both GDP- and GTP-bound forms of Rab9 ( Fig. 4l ), it appears that GFP-Rab9-S26N recruits Vps35 to the endosomal membrane but failed to concentrate it to the membrane budding site. Rab7 is known to recruit the retromer complex to LEs [38] , [39] . Downregulation of Rab7 prevented the accumulation of Vps35-mRFP in the budding structures ( Supplementary Fig. S4k ). Notably, Vps35-mRFP was often found inside endosomes (yellow arrowheads in Supplementary Fig. S4f , see also Supplementary Fig. S4k , showing a similar phenotype induced by a GDP-locked form GFP-Rab7-T22N), suggesting that the blockade of Rab7 activity resulted in the missorting of Vps35-mRFP into the endosomal lumen. Taken together, the results indicate that Rab5, Rab9 and Rab7 act sequentially during early to late endosomal maturation to recruit Vps35 to the endosomal-budding site (see Discussion ). Sorting of Serp into actin-rich endosomal-budding sites Actin is vital for vesicles to bud off the endosome. We therefore wondered if actin constitutes a component of the vesicle-budding machinery for Serp retrieval. Phalloidin staining of S2 cells revealed intracellular puncta ( Fig. 6a ) that colocalized with Vps35-mRFP ( Fig. 6a ) and the budding structures on LEs labelled with GFP-Rab9 ( Fig. 6b ). The colocalization of actin at the GFP-Rab9-labelled endosomal-budding sites was also observed in tracheal cells at stages 15 and 16 (blue arrowheads in Fig. 6c ). Triple labelling with GFP-Rab9, Vps35-mRFP and phalloidin confirmed that they all colocalized at the endosomal-budding site (white arrowheads in Fig. 6e ). Importantly, the cargo Serp was also colocalized with the actin-enriched endosomal-budding site ( Fig. 6f ). These results led us to investigate the actin dynamics in the endosome membrane. We co-transfected S2 cells with actin filament marker lifeact-mEGFP, and RFP-Rab9, and observed that endosomal budding occurred at actin patches on the RFP-Rab9 endosomes ( Supplementary Movie 3 , Fig. 6g magenta and green arrowheads). Strikingly, actin appeared before formation of the budding vesicles (compare the green arrowheads with magenta ones in Fig. 6g ), suggesting that the recruitment of actin is a prerequisite for vesicle budding. GDP form of Rab7 ( Fig. 6h ) and Rab9 ( Fig. 6i ) did not impair the localization of actin puntca at the endosomal membrane, indicating that recruitment of actin patches is Rab7 and Rab9 independent. Taken together, these data indicate that Serp-containing vesicles leave the LEs using an actin-involved budding machinery. 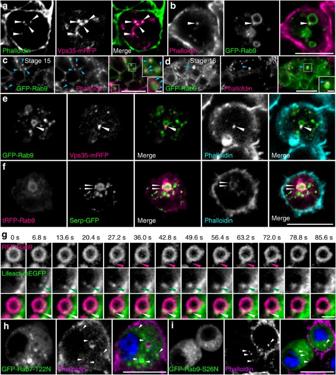Figure 6: Retrieval of Serp-containing vesicles from actin-enriched budding membranes of Rab9 endosomes. (a) Vps35-mRFP-expressing S2 cells stained with phalloidin. White arrowheads indicate the colocalization of actin patches with Vps35-mRFP-positive vesicles. (b) S2 cells expressing GFP-Rab9 stained with phalloidin. White arrowheads show actin localized to the protrusive domains of GFP-Rab9-labelled endosomes. (c,d) Embryos at the indicated stages expressingbtl-GAL4>GFP-Rab9 stained with phalloidin. Blue arrowheads in the insets indicate actin puncta localized to the protrusive domains of GFP-Rab9-labelled endosomes. (e) S2 cells co-transfected with GFP-Rab9 and Vps35-mRFP and stained with phalloidin. White arrowheads indicate GFP-Rab9, Vps35-mRFP and actin patch colocalized at the Rab9-enriched domain in GFP-Rab9-positive endosomes. (f) S2 cells expressing mRFP-Rab9 and Serp-GFP stained with phalloidin. White arrowheads indicate Serp-GFP puncta colocalized with actin patches in the Rab9 endosomal membrane. (g) Time-lapse images of endosomal budding in S2 cells co-expressing lifeact-mEGFP and RFP-Rab9, showing that actin is recruited to Rab9-positive endosome undergoing membrane budding and scission (Supplementary Movie 3). Magenta arrowheads indicate the protrusive membrane formation in Rab9 endosomes, and green arrowheads show the emergence of the actin patch earlier than membrane protrusion. White arrowheads indicate colocalization. (h,i) S2 cell expressing GFP-Rab7-T22N (h) and GFP-Rab9-S26N (i) stained with phalloidin. White arrowheads show actin puncta colocalized with endosomes. Scale bar, 10 μm fora–f,handiand 2 μm forg, insets incandd. Figure 6: Retrieval of Serp-containing vesicles from actin-enriched budding membranes of Rab9 endosomes. ( a ) Vps35-mRFP-expressing S2 cells stained with phalloidin. White arrowheads indicate the colocalization of actin patches with Vps35-mRFP-positive vesicles. ( b ) S2 cells expressing GFP-Rab9 stained with phalloidin. White arrowheads show actin localized to the protrusive domains of GFP-Rab9-labelled endosomes. ( c , d ) Embryos at the indicated stages expressing btl -GAL4>GFP-Rab9 stained with phalloidin. Blue arrowheads in the insets indicate actin puncta localized to the protrusive domains of GFP-Rab9-labelled endosomes. ( e ) S2 cells co-transfected with GFP-Rab9 and Vps35-mRFP and stained with phalloidin. White arrowheads indicate GFP-Rab9, Vps35-mRFP and actin patch colocalized at the Rab9-enriched domain in GFP-Rab9-positive endosomes. ( f ) S2 cells expressing mRFP-Rab9 and Serp-GFP stained with phalloidin. White arrowheads indicate Serp-GFP puncta colocalized with actin patches in the Rab9 endosomal membrane. ( g ) Time-lapse images of endosomal budding in S2 cells co-expressing lifeact-mEGFP and RFP-Rab9, showing that actin is recruited to Rab9-positive endosome undergoing membrane budding and scission ( Supplementary Movie 3 ). Magenta arrowheads indicate the protrusive membrane formation in Rab9 endosomes, and green arrowheads show the emergence of the actin patch earlier than membrane protrusion. White arrowheads indicate colocalization. ( h , i ) S2 cell expressing GFP-Rab7-T22N ( h ) and GFP-Rab9-S26N ( i ) stained with phalloidin. White arrowheads show actin puncta colocalized with endosomes. Scale bar, 10 μm for a – f , h and i and 2 μm for g , insets in c and d . Full size image WASH is essential for endosome abscission and Serp recycling WASH is a newly identified actin nucleation-promoting factor acting through its Arp2/3-interacting VCA domain (Verprolin homology, cofilin homology and acidic domain) [40] , having a critical role for endosomal vesicle budding in vitro [27] , [28] . To determine whether WASH is involved in Rab9 vesicle-budding process, we first showed that WASH expressed in the tracheal cells and colocalized with intracellular actin puncta labelled by lifeact-mEGFP ( Fig. 7a ). Then, we stained GFP-Rab9-expressing tracheal cells with WASH, and found that most of WASH puncta was localized at the Rab9 endosomal membrane (90%, n =8 cells Fig. 7b ). Double staining of WASH and Serp showed that WASH partly colocalized with intracellular Serp granules, which was contained inside Rab9 endosomes ( Fig. 7c ). WASH localized more proximal ( Fig. 7d ) than Vps35-mRFP ( Fig. 5b ) at the Rab9-enriched endosomal membrane. Actin patch was adjacent to WASH ( Fig. 7e ) and localized to the proximal part of Vps35-mRFP ( Fig. 6e ). To probe the function of WASH, we generated full-length and VCA domain-deleted dominant-negative [27] forms of GFP-WASH constructs, and transfected them into S2 cells with RFP-Rab9. The results showed that GFP-WASH formed puncta structures and localized at Rab9 endosomal membrane (white arrowheads in Fig. 7f ). GFP-WASH-ΔVCA can also localize on the endosomal membrane. However, long tubular structures were ectopically formed on endosomal membranes (white arrowheads in Fig. 7g ). In rab9 and vps35 mutant embryos, Association of WASH with Serp granules remained (white arrowheads in Fig. 7h ), indicating that the association of WASH and actin with cargo is independent of Rab9 and Vps35. In wash Δ185 -mutant [40] embryos, DT length was significantly longer than the control ( Fig. 7j–l ), and the luminal Serp level was reduced at stage 15 and later, phenocopying the Rab9- and Vps35-mutant phenotypes (white arrowheads in Fig. 7m ). The data collectively indicate that WASH, actin and Vps35 orderly localize to the budding site of Rab9 endosomal membrane, and constitute the major components of endosomal retrieval of Serp for recycling ( Fig. 7o ). 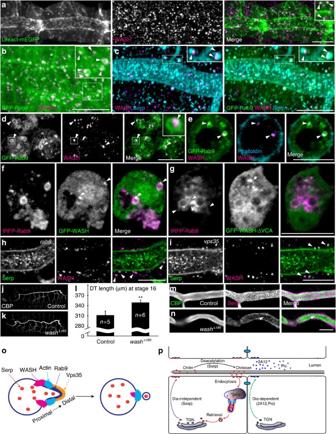Figure 7: WASH is required for tubular abscission and Serp recycling. (a) Tracheal cells expressing lifeact-mEGFP stained with WASH. White arrowheads in the inset indicate WASH colocalized with actin patches. (b) Tracheal cells expressing GFP-Rab9 stained with WASH. WASH localized at the Rab9 endosomal membrane. White arrowheads in the inset indicate one or two WASH puncta localized at one endosome. (c) Tracheal cells expressing GFP-Rab9 stained with WASH and Serp. Each intracellular Serp granule was associated with one or two WASH patches (white arrowheads in the inset inc). (d,e) S2 cells expressing GFP-Rab9 stained with WASH (d), and both phalloidin and WASH (e). WASH localized on Rab9-enriched subdomain of endosomal membrane (white arrowheads ind) and colocalized with actin puncta on the Rab9 endosomal membrane (white arrowheads ine). (f,g) S2 cells were co-transfected with RFP-Rab9, GFP-WASH (f) and RFP-Rab9, GFP-WASH-ΔVCA (g), respectively. Arrowheads infshow GFP-WASH puncta localized at the Rab9 endosomal membrane. White arrowheads ingshow the tubular and membrane cluster structures in Rab9 endosomes. (h,i)rab9-andvps35-mutant embryos stained with Serp and WASH, respectively. White arrowheads show that WASH puncta were associated with Serp granules inrab9-(h) andvps35-(i) mutant DT. (j,k) Control andwashΔ185-mutant embryos stained with CBP. (l) Quantification of DT length in control andwashmutation. Double (**) asterisks represent a significant difference betweenwashmutant and the control by Student’st-test (0.001<P<0.01). (m,n) Control andwash-mutant embryos stained by CBP and Serp. White arrowheads innshow decrease of Serp but not chitin expression in the lumen. (o) Composition and organization of retrieval machinery for vesicle budding. WASH, actin, Rab9 and Vps35 sequentially localize at the endosomal tubular structure. They constitute the main components of retrieval machinery for vesicle budding from endosomes. (p) Two major pathways of vesicle trafficking regulate luminal materials. At the late stage ofDrosophilatracheal development, the endocytosed luminal protein Serp is sorted into endosomal-budding membranes enriched with WASH, actin, Rab9 and Vps35, and recycled to the TGN for secretion by a Dia-independent pathway, whereas the secretion of other luminal markers, such as 2A12 and Pio, uses a Dia-dependent pathway. Thus, two distinct luminal protein trafficking pathways separately regulate tube morphogenesis. See text for details. Scale bar, 10 μm. Figure 7: WASH is required for tubular abscission and Serp recycling. ( a ) Tracheal cells expressing lifeact-mEGFP stained with WASH. White arrowheads in the inset indicate WASH colocalized with actin patches. ( b ) Tracheal cells expressing GFP-Rab9 stained with WASH. WASH localized at the Rab9 endosomal membrane. White arrowheads in the inset indicate one or two WASH puncta localized at one endosome. ( c ) Tracheal cells expressing GFP-Rab9 stained with WASH and Serp. Each intracellular Serp granule was associated with one or two WASH patches (white arrowheads in the inset in c ). ( d , e ) S2 cells expressing GFP-Rab9 stained with WASH ( d ), and both phalloidin and WASH ( e ). WASH localized on Rab9-enriched subdomain of endosomal membrane (white arrowheads in d ) and colocalized with actin puncta on the Rab9 endosomal membrane (white arrowheads in e ). ( f , g ) S2 cells were co-transfected with RFP-Rab9, GFP-WASH ( f ) and RFP-Rab9, GFP-WASH-ΔVCA ( g ), respectively. Arrowheads in f show GFP-WASH puncta localized at the Rab9 endosomal membrane. White arrowheads in g show the tubular and membrane cluster structures in Rab9 endosomes. ( h , i ) rab9- and vps35 -mutant embryos stained with Serp and WASH, respectively. White arrowheads show that WASH puncta were associated with Serp granules in rab9- ( h ) and vps35- ( i ) mutant DT. ( j , k ) Control and wash Δ 185 -mutant embryos stained with CBP. ( l ) Quantification of DT length in control and wash mutation. Double (**) asterisks represent a significant difference between wash mutant and the control by Student’s t -test (0.001< P <0.01). ( m , n ) Control and wash -mutant embryos stained by CBP and Serp. White arrowheads in n show decrease of Serp but not chitin expression in the lumen. ( o ) Composition and organization of retrieval machinery for vesicle budding. WASH, actin, Rab9 and Vps35 sequentially localize at the endosomal tubular structure. They constitute the main components of retrieval machinery for vesicle budding from endosomes. ( p ) Two major pathways of vesicle trafficking regulate luminal materials. At the late stage of Drosophila tracheal development, the endocytosed luminal protein Serp is sorted into endosomal-budding membranes enriched with WASH, actin, Rab9 and Vps35, and recycled to the TGN for secretion by a Dia-independent pathway, whereas the secretion of other luminal markers, such as 2A12 and Pio, uses a Dia-dependent pathway. Thus, two distinct luminal protein trafficking pathways separately regulate tube morphogenesis. See text for details. Scale bar, 10 μm. Full size image Maturation of the tracheal tube involves diameter expansion triggered by a cell-intrinsic programme of luminal material secretion and apical membrane growth [6] , [7] , and the tube’s longitudinal growth is negatively regulated by the presumed conversion of chitin to chitosan through deacetylation by chitin deacetylase [15] . Each step involves temporally regulated apical secretion, but the regulatory mechanism underlying this selective cargo secretion has not been understood. In this study, we identified Serp as a novel cargo for the Rab9-mediated retrograde recycling pathway. Using time-lapse imaging, we demonstrated that Serp in the endocytic compartment is sorted out by the budding of actin- and WASH-enriched portions of the LEs. The similarity of the Rab9, Vps35, WASH and Serp tracheal tube-length phenotypes, and the colocalization of those in the Serp-containing endosomal-budding sites in S2 cells, suggest that Serp is one of the major cargoes of the retrograde trafficking mediated by Rab9, Vps35 and WASH ( Fig. 7p ). We also found that association of WASH and actin filaments with retrograde cargo is Rab9 and Vps35 independent. Modular organization of machineries for cargo retrieval (retromer) and membrane remodelling (WASH) may allow flexibility in endosomal sorting systems. Our work connects retrograde trafficking to luminal retention of the key rate-limiting protein required to restrict the tracheal tube length to the proper level [15] , [16] and has identified a new regulatory process for tracheal tube size. Previous works in mammalian cells revealed that recruitment of the cargo recognition subcomplex of retromer (Vps35, Vps29 and Vps26) to the endosomal membrane requires Rab5 and Rab7 (refs 38 , 39 ). Rab7 has been shown to bind directly to Vps35/29/26 complex [38] , but no evidence is available for association of Rab5 or Rab9 with those components [38] , [39] . Our analysis of the Drosophila counterparts have shown that conversion of early to LE is accompanied by gradual reduction of relative abundance of GFP-Rab5 to RFP-Rab9 signals ( Supplementary Fig. S4 ). Throughout the process, Vps35-mRFP is present as distinct puncta associated with endosomes (yellow and white arrowheads in Fig. 5a ). We propose the following order of Rab9-Vps35 assembly. In early endosome, Rab9 recruits Vps35 to the endosomal membrane through physical binding. This process requires Rab5. After initial recruitment of Vps35, endosomal maturation proceeds with exchange of Rab5 with Rab7, which promotes retromer assembly and cargo concentration, followed by membrane scission induced by WASH and F-actin. Together, our results indicate that Rab5, Rab9 and Rab7 acts on retromer assembly at different stages of endosomal maturation and tubular membrane formation, where Serp and other cargos are retrieved for retrograde pathway ( Fig. 7o ). In contrast to the tracheal diameter expansion, which is triggered by a cell autonomous burst of exocytosis [6] , [7] , axial elongation is a slow and continuous process spanning stage 14–16. Therefore, any mechanism that restricts elongation is expected to be active throughout the elongation process. Previous studies showed that the two chitin deacetylases Serp and Verm act additively in tube length control [15] , [16] and the overexpression of either one causes the same tube length defects [16] , indicating that the amount of luminal chitin deacetylase must be precisely maintained. Furthermore, the expression of Serp mRNA in the trachea declines at stage 16 (ref. 15 ), when luminal Serp protein is still abundant ( Fig. 2b ), implying that Serp synthesized in the previous stage must be effectively retained and reused. Here we have shown that Serp is endocytosed and associates with GFP-Rab9 ( Fig. 2 ). The requirement for Rab9 and Vps35 for the luminal retention of Serp suggests that the endocytosed Serp is sorted from LEs to the TGN for secretion into the lumen, and this recycling pathway actively maintains the steady-state level of Serp to optimize the tube elongation process. Moreover, the retrieval transport through the TGN might help promote the modification of the endocytosed Serp, to recover its activity or to bind to an adaptor for its subsequent polarized secretion [41] . In rab9 , vps35 and wash mutants, Serp was mislocalized at the apical cortex of tracheal cells. This mislocalization may have been due to the trapping of Serp in endosomes marked with Rab7 or Rab11 which are apically localized in a Rab9-independent manner ( Supplementary Fig. S2g–j ). Consistent with this idea, a recent report showed that the suppression of Vps35 expression in NLT cells and neurons causes the accumulation of its cargo protein β-secretase (BACE1) in endosomes [42] . The second possibility is that the loss of Rab9 diverts the trafficking route of Serp from the endosomes to the cell surface, as observed in Rab9-deficient HeLa cells [43] . In support of this idea, we observed an enhancement of Serp accumulation at the surface of the epidermis in rab9 mutants (yellow arrowheads in Supplementary Fig. S2k,l ). The third possibility is that a defect in endocytosis arrested Serp at the apical membrane, because Vps35 has been shown to be involved in endocytosis in S2 cells [44] . Further analysis will be required to understand the diverse influences of retrograde trafficking on endosomal dynamics. The apical localization of Crb depends on the retromer complex [29] , [30] , but it was unaffected in rab9 mutants ( Supplementary Fig. S2 ). One possible explanation for this finding is that the alternative recycling pathway of Crb, which involves Rab11 [45] , compensates for the defect in retrograde trafficking in rab9 mutants. Another possibility is that Crb-retromer and Serp-retromer complexes use different trafficking pathways distinguished by sorting nexins [46] , [47] , which organize endosomal membranes into distinct morphological and functional regions for transport to diverse destinations [47] , [48] , [49] . Further study of the different sorting nexins should uncover the role of Rab9 in retromer cargo specificity. The Dia and motor protein Myosin V were shown to be required for the secretion of a number of markers, including 2A12 antigen, Pio and artificial ANF-GFP, into the tracheal lumen [8] . On the other hand, the secretion of Serp and Verm and the cell-surface localization of Crb are normal in Dia mutants, indicating that a Dia-independent secretory pathway regulates these protein localizations in the trachea [8] . The spectrum of secreted protein localizations affected in the rab9 and vps35 mutants was nearly complementary to that of Dia, suggesting that the Dia-dependent and retrograde trafficking-dependent mechanisms are the two major apical secretory pathways in the trachea ( Fig. 7p ). Verm localization was not affected in the rab9 and vps35 mutants, suggesting that this putative chitin deacetylase behaves differently from Serp [50] . The difference in cargo specificity for each pathway allows cells versatility in controlling the localization of different proteins according to distinct schedules, so that the secretory burst that triggers tube diameter expansion and the continuous recycling of chitin deacetylases in axial elongation are controlled separately. Our results provide a molecular basis for the roles of distinct trafficking pathways in controlling tubule growth and geometry. Fly strains and genetics rab9 deletion mutations were generated using Minos transposon imprecise excision [37] . Three lethal deletions ( rab9 56 , rab9 199 and rab9 366 ) were identified from 540 progenies. The region of each mutant encompassing the deletion was PCR amplified using genomic DNA from homozygous mutant embryos with the following primer pairs: rab9 56 , forward (f): 5′-CTGATGTTTAAGGCTAGTGCCTGC-3′, reverse (r): 5′-TGCAAGACTCAAAAACGTGTC-3′; rab9 199 , f: 5′-CCAATCGCTACGAGGAGAACAAC-3′, r: 5′-GAGCATCATTCCACGCTGTGTG-3′; and rab9 366 , f: 5′-TGAATGCGAGTGTTGACCTTGC-3′, r: 5′-CAATAGCGAAATCTGCCGAACCC-3′ The PCR products were subcloned into the pBluescript II KS vector for sequencing. rab9 56 , rab9 199 , rab9 56 /rab9 199 and rab9 366 showed similar tracheal tube length phenotypes; dvps35 1 was a kind gift from Xinhua Lin [31] ; the vps35 rab9 double mutant was generated by crossing recombination. vps35 1 rab9 56 , vps35 1 rab9 199 and vps35 1 rab9 366 showed similar tracheal tube-length phenotypes. Other strains used in this study included: wash Δ185 , UAS-GFP-Rab5, UAS-YFP-Rab7, UAS-GFP-KDEL, UAS-GFP-LAMP1, Df(2L)Exel8041, Mi{ET1}Rab9MB05612 and sna Sco /SM6a P{hslLMiT}2.4 (all from the Bloomington Stock Center), UAS–galactosyltransferase (GalT)-CFP (a kind gift from Akiko Satoh, Hiroshima University), UAS-myc-Dvps35 (kindly provided by Xinhua Lin [31] ) and UAS-Serp-CBD-GFP (generously provided by Stefan Luschnig [15] ). btl -GAL4 was used to drive the expression of UAS transgenes in the tracheal system. Molecular biology Full-length rab9 cDNA was amplified using the primers Rab9- Eco RI (5′-GGGAATTCGATGACGAACATGCGGCCGCC-3′) and Rab9- Bgl II (5′-CCACCAATTATCGGCTATGAAGATCTCCC-3′). The PCR product was purified, digested and ligated to the C-terminus of EGFP (GFP) or tagRFP (RFP) and inserted into the pUAST vector to generate the pUAST-GFP-Rab9 and pUAST-RFP-Rab9 transgenes. pUAST-GFP-Rab9-S26N was generated by a point mutant kit (QuickChange). Full-length (1–499 aa) and truncated (1–394 aa, VCA domain deleted) WASH was amplified using a common 5′-terminal primer WASH5 Eco RI (5′-TACAGAATTCGATGGAGGAGTCACCTTACCTGCACA-3′) and two 3′-terminal primers WASH3 Not I (5′-TACAGCGGCCGCCTAGTTCCACCCATCCTCGTCGT-3′) and WASHΔVCA3 Not I (5′-TACAGCGGCCGCCTACTCAGATCGCGGATCTTCAGTAGC-3′). The purified PCR products were ligased into pUAST-EGFP-C vector to make pUAST-EGFP-WASH and pUAST-EGFP-WASHΔVCA constructs, respectively. pUAST-lifeact-mEGFP was constructed by the amplification of Lifeact-mEGFP from a previously described Gateway expression plasmid [51] using Lifeact- Xho I (5′-CCGCTCGAGCAACATGGGTGTCGCAGATTTGATCAAG-3′) and Lifeact-mEGFP- Xba I (5′-GCTCTAGATTACTTGTACAGCTCGTCCATGCC-3′), and the insertion of the digested product into the pUSATattB vector. All the constructs were confirmed by DNA sequencing. Transgenic strains were established by DNA microinjection. The pUAST-Serp-GFP plasmid was provided by Stefan Luschnig [15] ; pUASp-GFP-Rab7, pUASp-GFP-Rab7-T22N and pUASp-GFP-Rab5 were kindly given by Tsubasa Tanaka and Akira Nakamura [52] ; UAS-myc-Dvps35 was a gift from Xinhua Lin [31] and pMT-blast-Vps35-mRFP was a kind gift from Cahir J O’Kane [44] . RNAi-induced gene knockdown Purified dsRNA products of Rab5, Rab7, Rab9, Vps35 and LacZ (control) were prepared according to the protocol previously described [53] . The primers used in the experiments were Rab5fw: 5′-TAATACGACTCACTATAGGGCGGTACCACAGCTTAGCTCC-3′ Rab5res: 5′-TAATACGACTCACTATAGGGGTTCGTCGGTCGATTTGTTT-3′ Rab7fw: 5′-TAATACGACTCACTATAGGGTTCCTCATACAGGCCAGTCC-3′ Rab7res: 5′-TAATACGACTCACTATAGGGGACAGTTGTCAGGATTGCCA-3′ Rab9fw: 5′-TAATACGACTCACTATAGGGGCGATTCCGGGCTCTACGCACCCCG-3′ Rab9res: 5′-TAATACGACTCACTATAGGGTCGGCCACGCACTCCATGTGCC-3′ Vps35fw: 5′-TAATACGACTCACTATAGGGGGCAAAGGCTAAAGCATGTCCTA-3′ Vps35res: 5′-TAATACGACTCACTATAGGGCTTTCCACTCCAGAAAAGCGC-3′ LacZfw: 5′-TAATACGACTCACTATAGGGGCATAAACCGACTACACAAATCAG-3′ LacZres: 5′-TAATACGACTCACTATAGGGGGCTTCATCCACCACATACA-3′. A total of 15 μg dsRNAs were added into 1 ml serum-free culture media for 45 min, then 2 ml normal S2 cell culture media containing serum was added into the wells and culture at 25 °C. After 72 h, the half cells were fixed for observation, another half was used for reverse transcription PCR to monitor the gene expression. Total RNA was prepared by using RNeasy mini kit (Qiagen) and RNase-Free DNase Set (Qiagen). Reverse transcription and PCR amplification were performed using SuperScript one-step reverse transcription PCR (Invitrogen). rp49 was chosen as internal control and the primers were as following: rp49_F: 5′-ATGACCATCCGCCCAGCATACAGG-3′ and rp49_R: 5′-TCGTTCTTCTTGAGACGCAGGCGA-3′. Cell culture, transfection and immunostaining Drosophila Schneider cells (S2 cells) were cultured in Schneider’s Insect Medium (Gibco) supplemented with 10% fetal calf serum and antibiotics at 25 °C. pUAS-vectors were co-transfected with actin5c-GAL4 drivers using Effectene (Qiagen) according to the manufacturer’s instructions. The expression of pMT-Vps35-mRFP was induced with 1 mM CuSO 4 overnight. After 24–48 h, the transfected cells were fixed and immunostained following previously described procedures [54] . GST pull-down experiment pGEX, pGEX-Rab7 (gift from Akira Nakamura) and pGEX-Rab9 were expressed in Escherichia coli BL21, and protein expression was induced with 0.1 mM IPTG for 16 h at 20 °C. GST-Rab recombinant proteins were purified by glutathione-sepharose 4B beads (Amersham). GST and GST-Rab proteins were immobilized on glutathione-sepharose 4B beads, then loaded with GDP or GTPγS following the previously described procedures [55] . UAS-myc-Vps35 was expressed in S2 cells for 48 h. The cells were collected and lysed in buffer containing 50 mM Tris–HCl, pH7.5, 150 mM NaCl, 5 mM MgCl 2 and 0.5% NP-40 for 30 min at 4 °C. Lysates were centrifuged and the supernatant was incubated with GST and GDP- or GTPγS-loaded GST and GST-Rabs for 2 h at 4 °C. The samples were subsequently washed five times with lysis buffer and eluted using SDS sample buffer and analysed by SDS–PAGE, immunoblotted with Mouse monoclonal anti-myc-HRP-DirecT and detected with ECL prime western blotting detection reagent (GE Healthcare). In situ hybridization Full-length rab9 cDNA was cloned into the pBluescript II KS vector and then digested with Xho I or Eco RI to create the template for in vitro transcription using T7 and T3, respectively, to produce sense and antisense probes for hybridization. Whole-mount wild-type and rab9 -mutant embryos collected 14–15 h after egg laying at 25 °C were fixed using 4% paraformaldehyde in PBS. rab9 -mutant homozygous embryos were collected from rab9 56 , rab9 199 or rab9 366 balanced over the Cyo-Dfd-YFP fly. In situ hybridization was conducted using digoxigenin (DIG)-labelled sense and antisense probes, according to a standard protocol [56] . Immunofluorescence staining and western blotting The primary antibodies used in this study were: mAb directed against Crb protein (1:40) (Developmental Studies Hybridoma Bank (DSHB)); mAb 2A12 antigen (1:2) (DSHB); rabbit anti-Pio (1:100), a gift from Markus Affolter [57] ; rabbit anti-Serp (1:300 and 1:1,000 for immunofluorescence and western blotting, respectively) and rabbit anti-Verm (1:300) generously provided by Stefan Luschnig [15] ; guinea pig anti-Uninflatible (1:500) was a gift from Robert E Ward [58] ; rabbit anti-Rab11 (1:8,000) and rabbit anti-Rab7 (1:3,000) were a kind gift from Tsubasa Tanaka and Akira Nakamura [52] ; CBP (1:200); phalloidin (1:100); WASH (1:50) [59] (DSHB); alpha-tubulin (DM1A) (1:8,000 for western blotting); and mouse monoclonal anti-Myc-HRP DirecT (1:5,000 for western blotting) (MBL). We were not able to obtain anti-Rab9 antibody that can be used for tissue staining, despite repeated attempts in raising polyclonal antibodies in mice and guinea pigs. For western blotting, 20 embryos were homogenized in loading buffer and heated for 10 min at 95 °C. The samples were loaded on 10% polyacrylamide gels for SDS-PAGE, and the proteins were transferred to polyvinylidene difluoride membranes. Immunoblotting and the detection of HRP-conjugated second antibodies with an ECL detection kit (GE Healthcare) were performed according to the manufacturer’s instructions. Morphometric analysis and statistics The DT was analysed in fixed stage-16 embryos ( n =6–9) using CBP staining. The DT length and diameter were determined with ImageJ (NIH, http://rsbweb.nih.gov/ij/ ). The DT length was measured from the anterior in tracheal segment 1 to the junction of the DT and transverse connective in tracheal segment 10. The DT diameter measurements were performed on maximal projections of Z stacks. For each embryo, the DT diameter was determined as the average value of three independent measurements taken in the central region of tracheal segment 7. The DT length and diameter were expressed as the mean plus standard deviation (SD) Student’s two-sided unpaired t -test with equal variance was used to assess the statistical significance. How to cite this article: Dong, B. et al . Rab9 and retromer regulate retrograde trafficking of luminal protein required for epithelial tube-length control. Nat. Commun. 4:1358 doi: 10.1038/ncomms2347 (2013).